An optimized optogenetic clustering tool for probing protein interaction and function The Arabidopsis photoreceptor cryptochrome 2 (CRY2) was previously used as an optogenetic module, allowing spatiotemporal control of cellular processes with light. Here we report the development of a new CRY2-derived optogenetic module, ‘CRY2olig’, which induces rapid, robust, and reversible protein oligomerization in response to light. Using this module, we developed a novel protein interaction assay, Light-Induced Co-clustering, that can be used to interrogate protein interaction dynamics in live cells. In addition to use probing protein interactions, CRY2olig can also be used to induce and reversibly control diverse cellular processes with spatial and temporal resolution. Here we demonstrate disrupting clathrin-mediated endocytosis and promoting Arp2/3-mediated actin polymerization with light. These new CRY2-based approaches expand the growing arsenal of optogenetic strategies to probe cellular function. Protein–protein interactions underlie nearly all molecular and cellular processes. As such, tools and technologies allowing scientists to probe and control protein interactions have fundamentally advanced our understanding of molecular and cellular mechanisms. Methods for detecting protein–protein interactions such as yeast two-hybrid and co-immunoprecipitation [1] , [2] , [3] are commonly part of every experimental biologist’s toolkit and have led to numerous new discoveries. In addition to tools for detecting protein interactions, technologies for controlling protein function have been instrumental in advancing scientific discovery. Chemical genetic tools allowing inducible control of processes have been critical for dissecting complex biochemical and signalling events within cells [4] , [5] ; however, these tools can be expensive, difficult to deliver to and remove from cells, and have limited temporal and spatial resolution. Emerging optical tools allow much finer control and observation of cellular processes using light, an actuator that can be delivered immediately and with subcellular spatial resolution. Optogenetic actuators allow light control of specific processes such as neuronal firing [6] , [7] , but more general tools have also been developed to manipulate protein transcription, protein–protein interactions and a variety of other cellular biochemical events [8] . In previous work, we developed one such tool, a system using the Arabidopsis flavoprotein cryptochrome 2 (CRY2) and its interacting partner CIB1 to inducibly control protein interactions with light [9] . While these proteins do not interact in the dark, blue light absorption triggers a conformational change in CRY2, allowing binding to CIB1 that is reversible after several minutes ( t ½ ~5.5 min). When attached to diverse target proteins, the CRY2 and CIB1 modules allow tight light regulation of target protein activity [9] , [10] , [11] , [12] , [13] . Wild-type CRY2 clusters in nuclear bodies in the nucleus of plant and animal cells with light [14] , [15] , [16] , and light-dependent clustering of CRY2 has also been adapted for light control, where it has been used to stimulate [17] or inhibit [18] protein function. While clustering appears to be a broadly useful approach to inducibly modulate cell function, wild-type CRY2 clusters poorly on its own, requiring high local protein concentrations or association with a multivalent protein partner [18] to achieve robust clustering. Here we describe a new CRY2-based optogenetic module, ‘CRY2olig’, that can be used on its own to probe and detect protein interactions in live cells, as well as to perturb protein function with light. When stimulated by a pulse of light, CRY2olig undergoes rapid, reversible, and robust clustering within seconds, redistributing a majority of cytosolic protein into clusters in every cell illuminated. While wild-type CRY2 also clusters under certain conditions [17] , clustering of CRY2olig is dramatically enhanced, enabling an entirely new set of experimental approaches for probing cellular biochemistry that cannot be achieved with existing tools. In the manuscript, we describe a new optical approach, Light-Induced Co-clustering (‘LINC’), using CRY2olig to query protein–protein interactions. We demonstrate the use of this approach to study protein interaction dynamics in live cells, as well as to query interactions in situ within small (sub-micrometer) intracellular domains. In addition to use querying protein interactions, we also demonstrate that CRY2olig provides a powerful tool to transiently and reversibly control protein function with light. As a proof-of-principle demonstration of use, we apply this tool to optically disrupt clathrin-mediated endocytosis and stimulate Arp2/3-mediated actin polymerization in live cells. These general optogenetic approaches are modular and can be used with a wide variety of target proteins, providing a powerful means to probe protein function within living cells. While screening for CRY2 variants with longer signalling states in a yeast two-hybrid assay ( Supplementary Fig. 1 ), we identified CRY2olig, containing an E490G mutation that greatly enhances light-induced clustering of CRY2. When fused to the reporter mCherry (mCh) and expressed in mammalian cells, CRY2olig–mCh shows diffuse expression in the dark, but upon blue light exposure it undergoes massive clustering, redistributing a majority of protein in the cytosol and nucleus (70±15% of cytosolic protein) into large puncta within tens of seconds following a pulse of light ( Fig. 1a–c and Supplementary Movie 1 ). Rate of clustering is dependent on protein concentration, with half-maximal clustering time varying from 75 to 15 s ( Fig. 1c ). Clusters appear to coalesce more rapidly and remain fixed in the nucleus, compared with the cytoplasm ( Fig. 1a and Supplementary Movie 1 ), perhaps due to interaction with nuclear components [15] . Clustering is light dose-dependent and maximally induced with only a 6 ms 488 nm light pulse at 5% laser power, conditions much lower than those typically used to image green fluorescent protein (GFP) ( Fig. 1d ). After clusters form with light, they reversibly dissociate in the dark but can be restimulated by a second light application ( Fig. 1e ). The half-life of dissociation from clusters ( t ½ =23.1 min) is longer than that reported for wild-type CRY2 ( t ½ ~6 min) [17] , [18] , consistent with our identification of CRY2olig as a mutant with a longer signalling state. 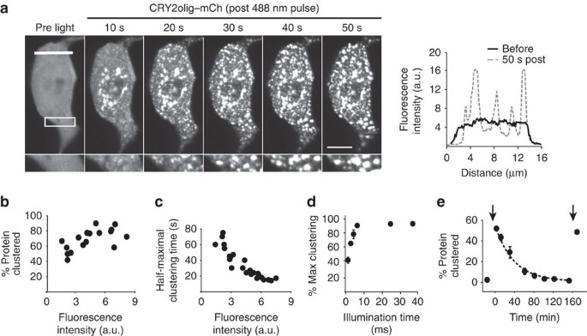Figure 1: CRY2olig undergoes rapid clustering with light. (a) HEK293 cells expressing CRY2olig–mCh pre and post blue light (25 ms pulse, 488 nm, 5% laser power). Graph at right shows the relative fluorescence intensity under the line in light versus dark. Scale bar, 7.5 μm. (b) Percentage of cytosolic CRY2olig–mCh depleted into clusters after light (25 ms pulse, 488 nm) correlated with mCh expression level (a.u.). (c) Graph showing dependency of half-maximal clustering time of CRY2olig–mCh on cellular expression level. (d) Light dose dependence. HEK293 cells expressing CRY2olig–mCh were exposed to 2.5–40 ms pulses of blue light (5% laser power), allowed to cluster, then illuminated with a saturating light pulse to induce maximal clustering. (e) Clustering recovery quantification. HEK293 cells expressing CRY2olig–mCh were exposed to light at timet=0 (first arrow), followed by a dark incubation for indicated times in the presence of 35 μg ml−1cycloheximide. A second pulse of light applied after recovery at 160 min (second arrow) induced re-clustering. Figure 1: CRY2olig undergoes rapid clustering with light. ( a ) HEK293 cells expressing CRY2olig–mCh pre and post blue light (25 ms pulse, 488 nm, 5% laser power). Graph at right shows the relative fluorescence intensity under the line in light versus dark. Scale bar, 7.5 μm. ( b ) Percentage of cytosolic CRY2olig–mCh depleted into clusters after light (25 ms pulse, 488 nm) correlated with mCh expression level (a.u.). ( c ) Graph showing dependency of half-maximal clustering time of CRY2olig–mCh on cellular expression level. ( d ) Light dose dependence. HEK293 cells expressing CRY2olig–mCh were exposed to 2.5–40 ms pulses of blue light (5% laser power), allowed to cluster, then illuminated with a saturating light pulse to induce maximal clustering. ( e ) Clustering recovery quantification. HEK293 cells expressing CRY2olig–mCh were exposed to light at time t =0 (first arrow), followed by a dark incubation for indicated times in the presence of 35 μg ml −1 cycloheximide. A second pulse of light applied after recovery at 160 min (second arrow) induced re-clustering. Full size image To directly compare clustering of CRY2olig with wild-type protein (CRY2PHR, containing the photosensory domain), we tested clustering under identical conditions in HEK293 cells ( Supplementary Fig. 2 and Supplementary Movie 2 ). In the dark, the proteins showed similar low levels of clustering (<1% of total protein clustered), with the majority of clusters forming in cells where the proteins were greatly overexpressed or concentrated (data not shown). In light, while only a small fraction (6±3%) of cytosolic protein in relatively few (12±7%) cells expressing CRY2PHR–mCh clustered (<1% of total cytosolic protein), ~40–90% of cytosolic CRY2olig–mCh redistributed into clusters in 100% of cells illuminated (~70% of total cytosolic protein; Supplementary Fig. 2a,b ). Thus, the E490G mutation enhances clustering in the cell population by nearly two orders of magnitude. The enhanced clustering capability of CRY2olig was not due to enhanced expression: all cells expressing CRY2olig, even at very low levels, showed clustering ( Supplementary Fig. 2c ). While it is possible that CRY2PHR forms smaller oligomers with light that cannot be resolved, these results indicate that the E490G mutation is a much more potent clustering module with enhanced dynamic range that opens up new possibilities for optogenetic applications. As our initial characterization of the E490G mutant ( Fig. 1 ) was in the truncated CRY2PHR domain, we also tested full-length CRY2 with the E490G mutation (CRY2oligFL). CRY2oligFL clusters with similar kinetics, but forms smaller puncta with less total protein redistributed ( Supplementary Fig. 3a,b and Supplementary Movie 3 ), suggesting that the C-terminal extension may restrict self-association. A CRY2olig–GFP fusion also clustered, as did untagged CRY2olig coexpressed with GFP–CIBN, a light-dependent interaction partner of CRY2 (refs 9 , 19 ) ( Supplementary Fig. 3c ), consistent with prior results showing CIB interacts with wild-type CRY2 clusters [17] , [18] . While we did not observe robust clustering of wild-type CRY2PHR–mCh on its own, CRY2PHR–mCh did strongly cluster when coexpressed with CRY2olig–GFP ( Supplementary Fig. 3d ), indicating it could be incorporated into CRY2olig clusters. Taken together, these results indicate that CRY2olig is sufficient to induce clustering by itself and that interacting proteins can be recruited into clusters. As with the CRY2/CIB interaction [9] , CRY2olig clustering could be stimulated by two-photon excitation at 850 nm ( Supplementary Fig. 3e ), making the technology amenable to in vivo or tissue slice preparations. Finally, CRY2olig was not toxic to COS-7 cells or within neurons ( Supplementary Fig. 4 ). Visualization of protein interaction dynamics As photoactivation clusters both CRY2olig and any interacting protein, we considered use of CRY2olig to probe protein–protein interactions. Such a strategy, in which an interaction is assessed by inducing redistribution of one protein, and querying whether a second protein also redistributes, was used previously [20] , [21] . However, while previous approaches require chemicals (or chemicals plus light) to induce redistribution, our ‘LINC’ assay requires only light. As shown in Fig. 2a , a CRY2olig-tagged ‘bait’ protein and a fluorescent-tagged (FP-tagged) ‘prey’ are coexpressed. The prey is imaged prior to and post blue light application, which clusters the CRY2olig-bait. The prey co-clusters with the bait only if the proteins interact. 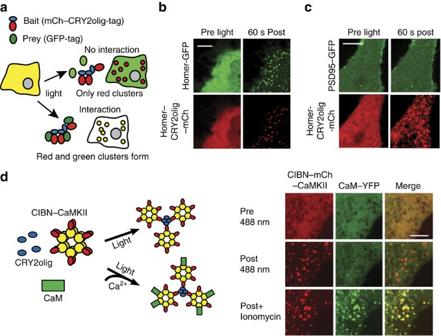Figure 2: LINC co-clustering assay to detect protein interactions. (a) Schematic describing LINC. (b) Positive control. COS-7 cells expressing homer1c–GFP co-cluster with homer1c–CRY2olig–mCh with blue light (50 ms pulse, 488 nm). Scale bar, 7.5 μm. (c) Negative control. PSD95–GFP does not co-cluster with homer1c–CRY2olig–mCh. Scale bar, 7.5 μm. (d) Assessment of dynamic interactions between CaMKII and CaM in response to Ca2+. COS-7 cells expressing CIBN–mCh–CaMKII, CRY2olig and CaM–YFP were imaged pre and post blue light exposure (500 ms pulse, 488 nm). At resting Ca2+, only a small amount of CaM–YFP colocalizes with CaMKII clusters. Addition of ionomycin elevates intracellular Ca2+, resulting in increased CaM–YFP localized to clusters. Scale bar, 5 μm. Figure 2b shows a proof-of-concept LINC experiment, demonstrating co-clustering of mCh and GFP-tagged versions of homer1c, a synaptic protein that homodimerizes [22] . In contrast, homer1c does not co-cluster with postsynaptic density protein 95 (PSD95), another synaptic protein that does not interact ( Fig. 2c ). LINC also works with membrane proteins, which are difficult to analyze by traditional methods, as demonstrated by co-clustering of stargazin and PSD95, two interacting membrane-associated proteins [23] ( Supplementary Fig. 5 and Supplementary Movie 4 ). Figure 2: LINC co-clustering assay to detect protein interactions. ( a ) Schematic describing LINC. ( b ) Positive control. COS-7 cells expressing homer1c–GFP co-cluster with homer1c–CRY2olig–mCh with blue light (50 ms pulse, 488 nm). Scale bar, 7.5 μm. ( c ) Negative control. PSD95–GFP does not co-cluster with homer1c–CRY2olig–mCh. Scale bar, 7.5 μm. ( d ) Assessment of dynamic interactions between CaMKII and CaM in response to Ca 2+ . COS-7 cells expressing CIBN–mCh–CaMKII, CRY2olig and CaM–YFP were imaged pre and post blue light exposure (500 ms pulse, 488 nm). At resting Ca 2+ , only a small amount of CaM–YFP colocalizes with CaMKII clusters. Addition of ionomycin elevates intracellular Ca 2+ , resulting in increased CaM–YFP localized to clusters. Scale bar, 5 μm. Full size image One advantage of LINC is that light may be applied at any time, allowing visualization of dynamic changes in interactions in response to a stimulus. To examine this, we visualized the interaction between Ca 2+ /calmodulin-dependent protein kinase II (CaMKII) and calmodulin (CaM), which is dependent on Ca 2+ (ref. 24 ; Fig. 2d ). Initial fusions of CaMKIIα to CRY2olig or even CRY2PHR resulted in substantial pre-clustering in the dark (data not shown), likely because CaMKII forms dodecamers that increase the propensity for CRY2 self-association. As an alternate means to cluster CaMKII, we tethered CaMKII to CIBN, which can be recruited into CRY2olig clusters. When coexpressed with CRY2olig and CaM–yellow fluorescent protein (CaM–YFP) and illuminated with blue light, CIBN–mCh–CaMKIIα clustered, but very little CaM–YFP colocalized ( Fig. 2d , post 488 nm).Addition of the Ca 2+ ionophore ionomycin prior to blue light clustering resulted in robust colocalization of CaM–YFP with CaMKII clusters. In addition to use with overexpressed FP-tagged proteins, we also show that LINC can be combined with immunofluorescent staining to detect endogenous CaM protein co-clustering with CaMKII ( Supplementary Fig. 6 ). LINC–FRAP assay to query interactions at compact sites While many assays can probe interactions in heterologous cells, fewer allow study of protein interaction dynamics in situ . To interrogate protein interactions in compact macromolecular structures (such as synapses, adherens junctions and kinetochores) where resident proteins already appear punctate, we extended LINC for use with Fluorescence Recovery After Photobleaching (FRAP) [25] . In ‘LINC–FRAP’, we also coexpress a CRY2olig-tagged bait and FP-tagged prey, but rather than assessing a change in localization of the FP–prey with light, we use FRAP to monitor the exchange rate and mobile fraction of the FP-tagged protein. The premise is that blue light will crosslink the CRY2olig-tagged bait, restricting its exchange, but also restricting the exchange of any interacting protein, which is assessed before and after exposure to blue light ( Fig. 3a ). 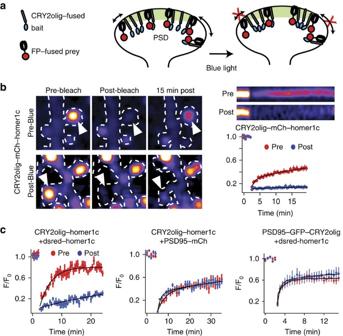Figure 3: LINC–FRAP assay. (a) Schematic describing use of LINC–FRAP in synapses. Mobility of a CRY2olig-fused protein (blue) is restricted after light-induced clustering, which restricts the mobility of an interacting FP-tagged protein (red). (b) LINC–FRAP control experiments in primary neuronal cultures showing exchange of CRY2olig–mCh–homer1c is delayed at the indicated photobleached synapse (arrowhead) after blue light clustering. (c) LINC–FRAP quantification before and after blue light, testing homer/PSD95 and homer/homer interactions at synapses. Figure 3: LINC–FRAP assay. ( a ) Schematic describing use of LINC–FRAP in synapses. Mobility of a CRY2olig-fused protein (blue) is restricted after light-induced clustering, which restricts the mobility of an interacting FP-tagged protein (red). ( b ) LINC–FRAP control experiments in primary neuronal cultures showing exchange of CRY2olig–mCh–homer1c is delayed at the indicated photobleached synapse (arrowhead) after blue light clustering. ( c ) LINC–FRAP quantification before and after blue light, testing homer/PSD95 and homer/homer interactions at synapses. Full size image We used LINC–FRAP to examine interactions within the PSD of neuronal synapses, small subcellular regions with an average diameter near the diffraction limit of light (~0.1–0.5 μm) ( Fig. 3 ). We first established that CRY2olig–mCh–homer1c rapidly exchanges at synapses before blue light exposure, but exchange is restricted after blue light ( Fig. 3b ). When CRY2olig–homer1c is coexpressed with DsRed–homer1c, DsRed–homer1c also exchanges rapidly prior to blue light. Rate of exchange at synapses is similar to that previously observed with an enhanced GFP (EGFP)-tagged homer1c [26] . After blue light exposure, exchange of DsRed–homer1c is severely limited, indicating interaction ( Fig. 3c ). In contrast, clustering of CRY2olig–homer1c does not affect the mobile fraction of PSD95–mCh, and clustering of PSD95–CRY2olig does not affect the mobile fraction of DsRed–homer1c ( Fig. 3c ), indicating that clustering one PSD resident protein does not generally restrict exchange of all PSD proteins. As interactions can be queried at different times, this method also enables study of interaction changes after a stimulus. These results demonstrate that LINC–FRAP will be a powerful tool to study the protein interaction landscape within compact subcellular domains in living cells. Transient perturbation of protein function using CRY2olig Given the dramatic redistribution of CRY2olig with light, we hypothesized that CRY2olig could be used not only to detect protein interactions, but also to acutely perturb them. While we were preparing this manuscript, another group independently demonstrated the use of CRY2 clustering to disrupt activity [18] , but the authors were unable to directly cluster targets fused to wild-type CRY2: clustering was induced by recruiting wild-type CRY2 to a second CIB-fused multivalent protein. In our case, we directly fuse CRY2olig to a target protein to allow inducible loss of function. As a proof-of-principle, we tested clathrin light chain (CLC), involved in endocytosis. Previously, crosslinking CLC using chemical dimerizers resulted in a ~70% inhibition of clathrin function [27] . We reasoned that tethering CLC to CRY2olig would allow conditional disruption of endocytosis with light ( Fig. 4a ). To assay endocytosis, we measured uptake of transferrin, which is internalized via clathrin-dependent endocytosis [28] . In COS-7 cells, CRY2olig–mCh–CLC clustered with light and showed a ~60% reduction in transferrin uptake in light compared with dark or untransfected cells ( Fig. 4b–d ). Disruption of endocytosis was reversible, as cells exposed to blue light followed by a 3 h dark incubation showed only a slight reduction in uptake ( Fig. 4d ). Using total internal reflection fluorescence (TIRF) microscopy, we visualized clathrin pit dynamics at the plasma membrane. Prior to blue light treatment, CRY2olig–CLC puncta colocalized with endocytic markers ( Supplementary Fig. 7 ) and underwent similar levels of dynamic events (appearing or disappearing from the surface) as a DsRed–CLC control ( Fig. 4e ). With light, we saw a reduction in dynamic events, similar to what was previously observed with chemical crosslinking [27] . The overall fluorescence intensity of clathrin pits also increased dramatically after light exposure ( Fig. 4f,g ), suggesting that cytosolic CRY2olig–CLC subunits were recruited to CRY2olig–CLC within clathrin pits, disrupting the precise architecture of these structures. 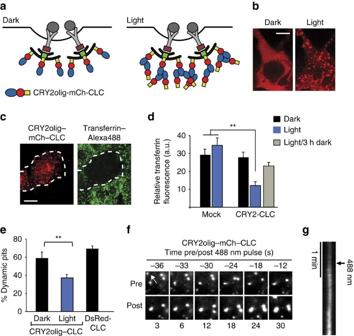Figure 4: Light-mediated disruption of clathrin-dependent endocytosis. (a) Schematic indicating light-mediated disruption of CLC function. (b) COS-7 cells expressing CRY2olig–mCh–CLC before and after blue light. Scale bar, 7.5 μm. (c) COS-7 cell expressing CRY2olig–mCh–CLC (inside dashed line) after exposure to blue light is defective for uptake of Alexa 488-transferrin (green), while surrounding untransfected cells show efficient uptake. Scale bar, 7.5 μm. (d) Quantification of transferrin uptake in untransfected (mock) versus CRY2olig–CLC-expressing cells exposed to dark, blue light or light/3 h dark. Data represents average and s.e.m.,n=15. **P<0.01. (e) Quantification of clathrin-coated pit dynamics within cells expressing CRY2olig–mCh–CLC in dark or after blue light (200 ms pulse, 488 nm), compared with a DsRed–CLC control. Data represents average and s.e.m.,n=3 cells (over 30 clusters per cell counted). **P<0.01. (f) TIRF images of COS-7 cells expressing CRY2olig–mCh–CLC, showing clathrin pits at the cell surface before and after blue light exposure (488 nm, 350 ms). Arrow indicates mobile clathrin pit undergoing endocytosis. (g) Kymograph of CRY2olig–mCh–CLC-labeled clathrin pit showing increase in fluorescence after light exposure. Figure 4: Light-mediated disruption of clathrin-dependent endocytosis. ( a ) Schematic indicating light-mediated disruption of CLC function. ( b ) COS-7 cells expressing CRY2olig–mCh–CLC before and after blue light. Scale bar, 7.5 μm. ( c ) COS-7 cell expressing CRY2olig–mCh–CLC (inside dashed line) after exposure to blue light is defective for uptake of Alexa 488-transferrin (green), while surrounding untransfected cells show efficient uptake. Scale bar, 7.5 μm. ( d ) Quantification of transferrin uptake in untransfected (mock) versus CRY2olig–CLC-expressing cells exposed to dark, blue light or light/3 h dark. Data represents average and s.e.m., n =15. ** P <0.01. ( e ) Quantification of clathrin-coated pit dynamics within cells expressing CRY2olig–mCh–CLC in dark or after blue light (200 ms pulse, 488 nm), compared with a DsRed–CLC control. Data represents average and s.e.m., n =3 cells (over 30 clusters per cell counted). ** P <0.01. ( f ) TIRF images of COS-7 cells expressing CRY2olig–mCh–CLC, showing clathrin pits at the cell surface before and after blue light exposure (488 nm, 350 ms). Arrow indicates mobile clathrin pit undergoing endocytosis. ( g ) Kymograph of CRY2olig–mCh–CLC-labeled clathrin pit showing increase in fluorescence after light exposure. Full size image We next examined whether CRY2olig could also be used to induce processes that are naturally stimulated by clustering. In one such example, antibody-mediated clustering of Nck SH3 domains resulted in localized induction of actin polymerization [29] . Using a similar approach, we fused the three SH3 domains of Nck to CRY2olig to generate CRY2olig–mCh–Nck, which showed diffuse localization in the dark but clustered with blue light ( Fig. 5a,b ). Actin clusters that colocalized with Nck clusters formed within seconds after light exposure ( Fig. 5b and Supplementary Movie 5 ), as did clusters of Neuronal Wiskott–Aldrich Syndrome protein (N-WASP) and N-WASP interacting protein, involved in Nck-mediated actin polymerization [30] , [31] ( Supplementary Fig. 8 ). In some cases, actin polymers could be observed that spanned NCK clusters (inset, Fig. 5b ). With prolonged light (>1 h), COS-7 cells expressing CRY2olig–Nck began to round up and lose their membrane extensions. To determine if local actin reorganization due to Nck clustering induced this phenotype, possibly by disrupting focal adhesion–actin connections, we locally photostimulated CRY2olig–Nck in cell extensions ( Fig. 5c and Supplementary Movie 6 ), which triggered retraction. To test the generality of this approach, we induced clustering of a completely different target, the Verprolin-homology, Central, Acidic (VCA) domain of N-WASP. Oligomerization of VCA was previously shown to greatly stimulate the actin nucleating activity of Arp2/3 (ref. 32) [32] . Upon light application, we observed rapid formation of CRY2olig–mCh–VCA clusters that colocalized with GFP–actin ( Fig. 5d,e and Supplementary Movie 7 ) and could not be reproduced by substituting CRY2PHR ( Supplementary Fig. 9 ). 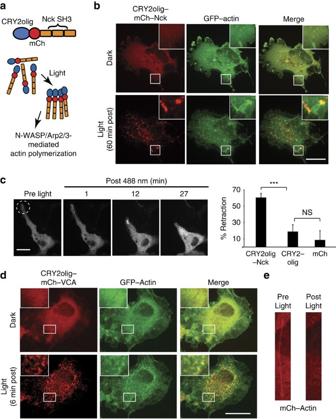Figure 5: Induction of actin cytoskeletal changes using CRY2olig. (a) Strategy for clustering Nck SH3 domains. (b) Cells expressing CRY2olig–mCh–Nck and GFP–actin in dark, or 60 min post blue light (500 ms pulse, 488 nm, every 3 min). Scale bar, 20 μm. (c) Local photostimulation (within circle) of COS-7 cell expressing CRY2olig–mCh–Nck results in retraction of cell extension. Graph at right shows quantification of retraction (average and s.e.m.,n=16) in cells expressing CRY2olig–mCh–Nck, or controls CRY2olig–mCh or mCherryN1 45 min post initial light exposure. ***P<0.001. NS, not significant. (d) Cells expressing CRY2olig–mCh–VCA, CRY2olig and GFP–actin in dark or 6 min post blue light (500 ms pulse, 488 nm, every 3 min). Inset images at right show detail within white square. Scale bar, 20 μm. (e) Stress fibres within cells expressing CRY2olig–GFP–VCA, CRY2olig and mCherry–actin are disrupted with light exposure. Figure 5: Induction of actin cytoskeletal changes using CRY2olig. ( a ) Strategy for clustering Nck SH3 domains. ( b ) Cells expressing CRY2olig–mCh–Nck and GFP–actin in dark, or 60 min post blue light (500 ms pulse, 488 nm, every 3 min). Scale bar, 20 μm. ( c ) Local photostimulation (within circle) of COS-7 cell expressing CRY2olig–mCh–Nck results in retraction of cell extension. Graph at right shows quantification of retraction (average and s.e.m., n =16) in cells expressing CRY2olig–mCh–Nck, or controls CRY2olig–mCh or mCherryN1 45 min post initial light exposure. *** P <0.001. NS, not significant. ( d ) Cells expressing CRY2olig–mCh–VCA, CRY2olig and GFP–actin in dark or 6 min post blue light (500 ms pulse, 488 nm, every 3 min). Inset images at right show detail within white square. Scale bar, 20 μm. ( e ) Stress fibres within cells expressing CRY2olig–GFP–VCA, CRY2olig and mCherry–actin are disrupted with light exposure. Full size image Here we introduce CRY2olig, a modular genetically encoded protein tag that can be used to inducibly trigger oligomerization of fused protein targets with light. We envision two broad uses for this tool in live cells: interrogating protein–protein interactions and perturbing protein function. As a tool for querying protein–protein interactions, the LINC technology has a number of advantages. LINC requires no major equipment beyond a fluorescent microscope, an instrument accessible to most researchers, and is relatively quick and easy to perform. The clustering phenotype is robust, thus interactions are scored without complex image analysis. As many labs already have numerous FP-tagged proteins available for use with other studies, these can be readily used as preys. Finally, protein interactions can be queried at user-defined timepoints in individual cells, allowing determination of how protein interactions change over time in response to a stimulus or inhibitory drug. The LINC–FRAP approach, used for probing interactions at compact intracellular sites, also provides advantages over previous methods. A similar FRAP approach was previously used to query interactions [33] , [34] , however, that method used antibodies to immobilize the bait proteins, and thus could only be used with transmembrane proteins. LINC–FRAP simplifies this approach (as light is used both to induce clustering and monitor mobility), and extends its use to intracellular proteins. The most versatile and commonly used technology for probing interactions in vivo at compact sites is Förster Resonance Energy Transfer (FRET), a powerful approach, but one that can be difficult to optimize for specific molecules and difficult to interpret since fluorophore crosstalk and differences in stoichiometry between labelled proteins can greatly influence outputs [35] . In contrast, LINC–FRAP requires little optimization. While LINC–FRAP does not provide a continuous readout of protein interaction dynamics such as can be achieved with FRET, by applying light at different times after a stimulus or treatment, changes in these interactions over time can be monitored. While LINC and LINC–FRAP have a number of advantages, we note that the technologies do not discriminate between direct and indirect protein–protein interactions. Co-clustering or co-immobilization can occur either between direct binding partners, or through an intermediate partner. In this sense, the technology is not different from co-immunoprecipitation or yeast two-hybrid, in which non-direct interactions are also a possibility. We also note that LINC does not allow verification of subcellular localization of interactions, as localization can potentially be altered by clustering. Finally, while this method as it stands is amenable to high-throughput screening using automated microscopy systems, we have not tested the use of this method with fluorescence-activated cell sorting-based sorting or other selection schemes. While we expect LINC and LINC–FRAP to be useful technologies, perhaps an even more powerful application of CRY2olig is the ability to control cellular function with light using a single, genetically encoded tag. While a number of different optical dimerizer systems for controlling the interactions of two proteins have emerged (see ref. 8 for a review), there remains an unmet need for optical tools to rapidly disrupt protein function that can be applied to any target. Because clustering triggered by CRY2olig is reversible, protein activity can be perturbed for precise user-defined periods of time. As light can be focally delivered to specific cells or even subcellular regions, CRY2olig can enable entirely new studies into spatial requirements of protein activity. For example, the CRY2olig–CLC tool may be used to study the consequences of blocking endocytosis at specific times within specific subcellular regions. In addition to disrupting protein function, we also show CRY2olig efficiently induces oligomeric-dependent processes. We demonstrate this by manipulating actin polymerization, a process known to be stimulated by clustering of Nck SH3 domains or the VCA domain of N-WASP. As we show in Fig. 5c , we can focally deliver light to induce clustering in a small region of the cell, thus enabling subcellular control of oligomeric-dependent processes. CRY2olig has advantages over other clustering tools such as antibody-mediated clustering [29] , [36] or chemical inducers of dimerization [37] , which require addition of chemicals or antibodies, have no spatial control and limited temporal control, and in the case of antibodies, can only be used with cell surface proteins. We also find CRY2olig to be a much more potent inducer of clustering than wild-type CRY2, which has been utilized to confer light control over signalling pathways stimulated by oligomerization [17] . For example, while we could induce actin reorganization with CRY2olig–VCA, we were unable to accomplish the same result using CRY2PHR–VCA ( Supplementary Fig. 9 ). Adding to its versatility, clustered CRY2olig retains interaction with CIB1, a light-dependent binding partner of wild-type CRY2, and thus can be used along with the CRY2/CIB system [9] for more complex control. While further studies are needed to address the precise mechanism of CRY2olig clustering—as CRY2 can dimerize in the dark, we hypothesize that light may induce a multivalent state and trigger a sol-gel phase transition [38] —ultimately, the strategies outlined here can be applied to any number of diverse targets to disrupt or stimulate protein activities with light, and to probe a variety of complex protein interactions. We anticipate that CRY2olig may be used in diverse ways to organize protein complexes within cells, for example, to assemble synthetic scaffolds of metabolic enzymes, allowing efficient substrate channelling through a metabolic pathway [39] , [40] . Given the growing recognition of the importance of scaffolding and compartmentalization in biology [41] , [42] , [43] , tools such as CRY2olig allowing rapid, reversible assembly or disruption of multi-protein complexes will enable a wealth of new studies. Generation of constructs CRY2olig consists of CRY2PHR (residues 1–498 of CRY2) containing a E490G mutation. Some constructs (noted below) also contain a second M354I mutation originally found with E490G, which does not appear to affect clustering or photoresponse. CRY2olig–mCh was generated by generating a E490G mutation in CRY2PHR–mCh [9] , containing CRY2PHR in the pmCherryN1 vector backbone (Clontech), using PCR with mutagenic oligos (5′-CTTGG CTC GAG GCC ACC ATG AAG ATG GAC AAA AAG ACT ATA GTT-3′) (5′-TCG ACC CCG TGC TGC TCC GAT CAT GAT CTG TGC TCC ACG GGT TCT TG-3′). The construct expressing CRY2olig (without a fluorescent tag) was generated by placing a stop codon at the end of the CRY2 domain of CRY2olig–mCh, before mCh. CRY2olig–GFP was generated by cloning CRY2olig (containing M354I) at XhoI—XmaI sites [9] into EGFP–N1 (Clontech). CIBN–GFP was generated by replacing the GFP–CAAX sequence in CIBN–pmGFP [9] with EGFP. CRY2oligFL–mCh was generated by PCR-based mutagenesis of CRY2–mCh (ref. 9 ) to add E490G. CRY2olig–mCh–CLC was generated by cloning CLC into a version of CRY2olig–mCh, containing residues CRY2 (with M354I) at BsrGI and NotI sites (5′-CGG TGT GTA CAA GTC CGG TGG AAT GGC CGA GTT GGA TCC ATT C-3′) (5′-GGA CCT GCG GCC GCT TAG TGC ACC AGA GGG GCC TG-3′). CRY2olig–mCh–Nck and CRY2olig–mCh–VCA were generated by amplifying either the SH3 domains of Nck (residues 1–258) (5′-GACG AGC TGT ACA AGG GAT CCA CCA TGG CAG AAG-3′) (5′-GAGTC GCG GCC GCT CAT TAA GC GTA ATC CGG AAC ATC GTA TGG GTA GGT ACC ACC TGA AGT TAA TGG ATT ATT CTG-3′) or the VCA domain of N-WASP (residues 388–501) (5′-CGG CGG CAT GGA CGA GC TGT ACA AGG GAT CCC CTT CTG ATG GTG ACC ATC-3′) (5′-CTAGA GTC GCG GCC GCT CAT TAA GCG TAA TCC GGA ACA TCG TAT GGG TAG GTA CCG TCT TCC CAC TCA TCA TCATC-3′) by PCR to add BsrGI and NotI restriction sites, then ligating into CRY2olig–mCh (containing M354I) cut with BsrGI and NotI. CRY2olig–mCh–CaMKIIα was cloned by digesting CRY2olig–mCh with NheI and BsrGI and ligating into a pEGFP (Clontech) backbone containing CaMKIIα. CIBN–mCh–CaMKII was generated by replacing CRY2olig in CRY2olig–mCh–CaMKII with CIBN at AgeI and NheI sites. DsRed–homer1c was generated by cloning homer1c at BsrGI and NotI sites into a vector containing the pcDNA3.1 backbone with dsRed inserted at the MCS. CRY2olig–mCh–homer1c was generated by cloning homer1c into CRY2olig–mCh (containing M354I) using BsrGI and NotI sites. PSD95–mCh was generated by cloning PSD95 into HindIII and EcoRI sites of mCherryN1 (Clontech). PSD95–mCh–CRY2olig was generated by amplifying CRY2olig (containing M354I) by PCR and cloning into PSD95–mCh at BsrGI and NotI sites (5′-GGT TAA TGT ACA GTG CTG GTA GTG CTG GTA GTG CTG GTA TGA AGA TGG ACA AAA AGACT-3′) (5′-AAT TAA GCG GCCGC TCA TGC TGC TCC GAT CAT GAT CTG-3′). Dynamin–mCherryN1 was obtained from Christien Merrifield (Addgene, plasmid 27697). TfR–SEP was described previously [44] . Yeast two-hybrid experiments GalBD plasmids containing CRY2PHR, a CRY2 mutagenic library (generated by error-prone PCR), or CRY2olig along with a pGADT7rec-CIB1 plasmid [9] were expressed in strain MaV203 ( MAT α leu2-3,112 trp-901 his3-200 ade2-1 gal4Δ gal80Δ SPAL10 -URA3 GAL1 -lacZ. LYS2:: GAL1 -HIS3 can1 R cyh2 R ). Yeast were grown at 30 °C for 72 h on SD–Trp/–Leu/–Ura under indicated light conditions (Dark; frequent light (1 s pulse every 3 min); Infrequent light (1 s pulse every 20 min). Illumination was applied using a 461 nm, 1.1 mW cm −2 light-emitting diode array. Live cell imaging HEK293 or COS-7 cells were cultured in Dulbecco's Modified Eagle's Medium (DMEM) with 10% foetal bovine serum, then seeded onto 18-mm coverslips or 35-mm glass bottom dishes (Mattek) in 12-well plates and transfected using Lipofectamine 2000 (Life Technologies) according to the manufacturer’s protocol. Cells were incubated in dark (wrapped with foil) and manipulations were carried out under dim light or using a red safelight. Twelve to twenty-four hours after transfection, cells were moved to Hepes-buffered Saline (HBS) with 1 mM CaCl 2 for imaging studies. Live cell imaging was performed at 33.5 °C on an Olympus IX71 microscope equipped with a spinning disc scan head (Yokogawa Corporation of America) with a × 60/NA 1.4 objective. Excitation illumination was delivered from an AOTF-controlled laser launch (Andor Technology) and images were collected on a 1,024 × 1,024 pixel EM-CCD camera (iXon; Andor Technology). For photoactivation studies ( Fig. 5c ), laser illumination (488 nm) was delivered using galvometric laser-scanning mirrors (FRAPPA; Andor Technology) at 1–2% of maximum power with a 100 μs dwell time. Two-photon excitation was performed on a Zeiss LSM510 microscope containing a Chamelon Ultra II laser (Coherent) tuned to 850 nm and 60% power with a 50 μs pixel dwell time. For light-sensitive experiments, cells were protected from ambient light sources by focusing in the presence of filtered light (572/28 bandpass filter, Chroma). Image analysis Data acquisition and analysis were performed using MetaMorph (Molecular Devices), ImageJ or Fiji. Per cent of protein in puncta was calculated by first determining the total fluorescence within puncta using manual ImageJ thresholding (Otsu’s method) to delineate protein within puncta contained with the cell cytosol. The total fluorescence within puncta was divided by the total fluorescence within each analyzed region. In some cases ( Fig. 1e ) to calculate protein in puncta, we also used ‘FindPeaks’ ( http://www.sussex.ac.uk/gdsc/intranet/microscopy/imagej/gdsc_plugins ), an ImageJ plugin, with the following parameters: background calculation, one s.d. above mean; autothreshold, Otsu method; minimum peak height relative above background, 0.10; minimum above saddle, 0.20. Comparison studies of CRY2PHR–mCh and CRY2olig–mCh For comparison studies, we transiently transfected CRY2PHR–mCh or CRY2olig–mCh into HEK293 cells, under identical conditions. After 24 h, we recorded time-lapse movies at random-sampled locations on the coverslip, recording an initial mCh image, followed by a GFP image that stimulated CRY2, followed by a mCh image series (every 30 s for 3 min). Fluorescence in puncta in dark and light were reported for sampled areas. Toxicity studies COS-7 cells were transfected with CRY2olig–GFP (in EGFP–N1 vector backbone) or EGFP–N1 (Clontech). Twenty hours after transfection, cells were kept in the dark or treated with light (1 s pulse, every 1 min, 461 nm, 1.1 mW cm −2 ) for indicated times. Twenty-four hours after the start of light treatment, propidium iodide (PI, Sigma, 2 μg ml −1 final concentration) was added to the media for 5 min then cells were washed with PBS. Cells stained with PI were manually counted on an Olympus CKX41 fluorescent microscope. For neuronal toxicity studies, primary hippocampal neurons were prepared from the hippocampi of neonatal Sprague–Dawley rats, dissected at postnatal day—0–2 rats—and dissociated by papain digestion. Neurons were plated at 60,000–70,000 cells per ml in MEM, 10% foetal bovine serum (Hyclone) containing penicillin/streptomycin on poly-d-lysine-coated glass coverslips. MEM media was replaced after 24 h with Neurobasal-A supplemented with B27 (Invitrogen). Neurons were incubated with Neurobasal-A, B27 and mitotic inhibitors (uridine+fluoro-deoxyuridine) by replacing half the media on day 4 or 5 and then twice weekly. Neurons were transfected on DIV 5–6 with Lipofectamine 2000 and imaged on DIV 6–7. One day after transfection, neurons were either kept in the dark or exposed to light (1 s pulse, every 1 min, 461 nm, 1.1 mW cm −2 ) for 3 min, then treated 24 h later with PI and quantified as described with COS-7 cells. All animal procedures were performed in accordance with the University of Colorado School of Medicine guidelines. LINC protein interaction studies LINC studies were carried out in COS-7 cells transiently transfected with indicated constructs. Cells were imaged before blue light exposure (with the ‘Dark’ GFP image initiating CRY2olig photoactivation) then every 10 s afterwards. COS-7 cells were transiently transfected with CIBN–mCh–CaMKII, unlabelled CRY2olig and CaM–YFP, and CaMKII clustering was induced by recruitment of CIBN into CRY2olig clusters. For ionomycin experiments, cells were incubated with 2 μM of ionomycin Ca 2+ salt for 1 min before light-induced clustering. For LINC–FRAP analysis at synapses, primary hippocampal neurons were prepared as described in ‘Neuronal toxicity studies’. Photobleaching of individual synapses was carried out using galvometric steered laser excitation (FRAPPA, Andor) at a single spot for 1 ms. Photobleaching pulses were calibrated so that they bleached no more than 50–75% of the original signal. Recovery was monitored following photobleaching every 15–60 s (depending on the recovery kinetics of the molecule under investigation). FRAP recovery rates were determined for different sets of synapses from the same neuron before and after blue light exposure. Quantification was performed using ImageJ. Immunocytochemistry COS-7 cells grown on coverslips were transiently transfected with CIBN–mCh–CaMKIIα and CRY2olig, then incubated the next day with 2 μM ionomycin for 1 min. Samples were either maintained in the dark or treated with blue light for 5 min (1 s pulse every 1 min, 461 nm, 1.1 mW cm −2 ). Cells were fixed with 4% paraformaldehyde for 10 min, permeabilized and blocked (PBS, 5% normal goat serum, and 0.1% triton X-100) for 1 h, then incubated with an α-calmodulin monoclonal antibody (1:50, 2D1, Pierce) followed by an α-mouse IgG AlexaFluor-488 secondary antibody (1:1,000, Jackson ImmunoResearch). Endocytosis studies COS-7 cells were seeded onto 18-mm coverslips, transfected with CRY2olig–mCh–CLC using Lipofectamine 2000, and incubated in the dark. Twenty-four hours after transfection, samples were either maintained in the dark or treated with blue light for 10 min (1 s pulse, every 1 min, 461 nm, 1.1 mW cm −2 ), followed by incubation with 50 μg ml −1 transferrin-AlexaFluor-488 (Life Technologies) for 10 min. Cells tested for dark recovery were exposed to 10 min of blue light pulses, then incubated in the dark for 3 h before transferrin labelling. After transferrin labelling, coverslips were washed in PBS and cells were fixed in 4% paraformaldehyde. For TIRF studies, we used an Olympus IX81 inverted motorized microscope equipped with laser illumination of 10 mW 488 nm argon, 543 nm HeNe coupled to a manual TIRF illuminator. A temperature of 34 °C was maintained throughout experiments. Images were recorded at 2 Hz on a CCD camera [Orca ER, Hamamatsu Photonics) using Slidebook software. Actin reorganization studies For global activation and clustering of CRY2olig–mCh–Nck and CRY2olig–mCh–VCA, CRY2olig was initally photoactivated by a 500 ms pulse of 488 nm laser illumination at 50% of maximum laser power, then imaged every 3 min afterwards for mCh and GFP. For local photoactivation, a ~15 μM-diameter region was photoactivated at the farthest tip of cell extensions and the change in cell extension area was quantified after 45 min. With VCA domain experiments, initial experiments using COS-7 cells expressing CRY2olig–mCh–VCA showed no light-dependent clustering, possibly due to steric effects of VCA fusions on CRY2 self-association. To circumvent this, we coexpressed CRY2olig–mCh–VCA along with unlabelled CRY2olig in a 1:1 ratio, so as to dilute any steric issues caused by CRY2olig–mCh–VCA: CRY2olig–mCh–VCA association. This strategy allowed clustering and was used for all VCA experiments. How to cite this article: Taslimi, A. et al. An optimized optogenetic clustering tool for probing protein interaction and function. Nat. Commun. 5:4925 doi: 10.1038/ncomms5925 (2014).